Principle of direct van der Waals epitaxy of single-crystalline films on epitaxial graphene There are numerous studies on the growth of planar films on sp 2 -bonded two-dimensional (2D) layered materials. However, it has been challenging to grow single-crystalline films on 2D materials due to the extremely low surface energy. Recently, buffer-assisted growth of crystalline films on 2D layered materials has been introduced, but the crystalline quality is not comparable with the films grown on sp 3 -bonded three-dimensional materials. Here we demonstrate direct van der Waals epitaxy of high-quality single-crystalline GaN films on epitaxial graphene with low defectivity and surface roughness comparable with that grown on conventional SiC or sapphire substrates. The GaN film is released and transferred onto arbitrary substrates. The post-released graphene/SiC substrate is reused for multiple growth and transfer cycles of GaN films. We demonstrate fully functional blue light-emitting diodes (LEDs) by growing LED stacks on reused graphene/SiC substrates followed by transfer onto plastic tapes. van der Waals epitaxy (vdWE) can allow crystalline growth on two-dimensional (2D) materials with no requirement to satisfy lattice mismatch between the growing materials and underlying 2D materials, resulting in reduced defect density [1] , [2] . Recently, this concept has drawn renewed attention with current substantial advancement of research on 2D layered materials [3] , [4] . If one can grow 2D blanket epitaxial films on 2D materials, it will open up a new opportunity to beyond current extensive research on large-scale fabrication of crystallographically aligned 2D heterostructures [3] , [4] . If one can grow sp 3 -bonded three-dimensional (3D) epitaxial films on 2D materials, it will allow transfer of single-crystalline semiconductor films due to weak van der Waals interaction between 2D materials and overlaying layers [5] . However, suppressed nucleation of adatoms on the surface of sp 2 -bonded 2D materials limits the large-area single-crystalline growth [2] , [6] , [7] , [8] , [9] , [10] . Therefore, most of the attempts to grow blanket films on 2D materials resulted in nonplanar film morphologies. For example, direct growth of 2D on 2D materials forms flakes such as MoS 2 flakes on graphene [2] , [11] , whereas direct epitaxy of sp 3 -bonded 3D materials on 2D materials causes the formation of 3D clusters such as GaN clusters on h-BN or graphene [2] , [6] , [7] , [8] , [9] , [10] . Recently, growth of planar 3D material films on 2D materials was demonstrated by employing interfacial buffers between 3D and 2D materials to promote nucleation of 3D materials on 2D materials such as GaN film growth on ZnO nanowalls/graphene [9] , [12] , [13] and GaN film growth on AlN/h-BN (or graphene) [10] , [14] . Even with the interfacial buffer, however, the quality of GaN films grown on 2D materials is significantly worse than that on a conventional SiC or sapphire substrate. In the best case, GaN on AlN/h-BN, the measured defect density (1.6 × 10 10 cm −2 ) is greater than that from conventional GaN epitaxial films grown on sapphire by more than one order of magnitude and surface roughness was not as low as that of conventional GaN epitaxial films on sapphire [10] , [15] . Having considering the fact that an AlN buffer has also been an essential component for conventional growth of high-quality GaN films on sapphire substrates [15] , different growth strategies are required for the epitaxy on 2D materials. Moreover, buffered growth is not applicable for the growth of 2D on 2D materials where direct contact of those materials makes device functions [3] , [4] and also for the growth of vertical electronic devices that require formation of initial films with high electrical conductivity [15] . Here we demonstrate direct growth of high-quality single-crystalline films on 2D materials. We choose epitaxial graphene grown on a SiC substrate as a template for growing single-crystalline films because it retains a unique orientation over an entire substrate and it contains the periodic nucleation sites at the step edges [16] , [17] . We perform direct vdWE of single-crystalline GaN films on epitaxial graphene on SiC substrates by careful control of growth kinetics. Even without using any buffer layers, GaN crystalline quality comparable with that typically obtained via conventional AlN-buffer-assisted GaN epitaxy on SiC or sapphire substrates is obtained by overcoming substantial lattice mismatch of ~23% between graphene and GaN. Measured root mean square (RMS) roughness is 3 Å and defect density is as low as 4 × 10 8 cm −2 . The entire high-quality single-crystalline GaN films are then released from the graphene and transferred on arbitrary substrates. Owing to precise release of GaN from the surface of graphene with no remaining GaN on the graphene, demonstration of multiple cycles of growth and transfer of GaN films is enabled by reusing the single graphene/SiC substrate with no requirement of post-release surface treatment. Additionally, thanks to the atomistic smoothness of released GaN surface, direct bonding of released GaN onto Si substrate is enabled. In this study, we introduce the epitaxial graphene as a reusable platform for multiple transfers of high-quality single-crystalline layers and offer the general principle of direct vdWE on 2D materials which may also be applicable to other materials systems such as 2D heterostructures. Graphene-based layer transfer graphene A schematic of our graphene-based layer transfer process is shown in Fig. 1 and the process consists of the following steps: formation of epitaxial graphene by self-limiting graphitization of a vicinal (0001) SiC substrate [16] , [17] ( Fig. 1a ), epitaxy of single-crystalline GaN films on graphene/SiC substrates by taking advantage of facilitated nucleation at vicinal steps ( Fig. 1b ), release of entire GaN films from the graphene surface by using a stressor metal (Ni) and the flexible handling layer (thermal release tape) [18] , [19] ( Fig. 1c,d ), transfer of the released GaN to host substrates ( Fig. 1e,f ) and multiple growths and transfers of the GaN films on/from the original graphene/SiC substrate. 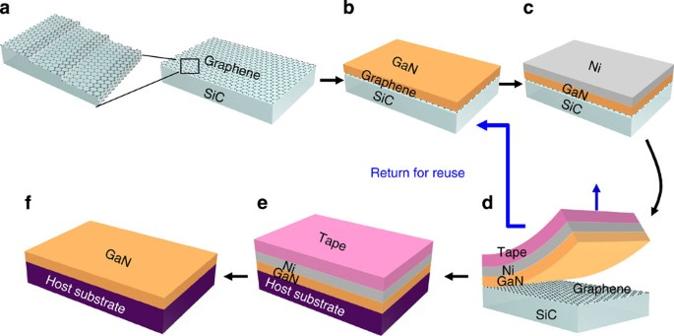Figure 1: Schematic of a method for growing/transferring single-crystalline thin films on/from epitaxial graphene. (a) Graphitization of a SiC substrate to form epitaxial graphene. (b) Epitaxial growth of GaN on graphene. (c) Deposition of a stressor layer (Ni). (d) Release of GaN from the substrate with a handling tape. (e) Transfer of the released GaN/Ni/tape stack on a host substrate. (f) Removal of the tape and Ni by thermal release and wet etching, leaving a GaN film on the host substrate. Figure 1: Schematic of a method for growing/transferring single-crystalline thin films on/from epitaxial graphene. ( a ) Graphitization of a SiC substrate to form epitaxial graphene. ( b ) Epitaxial growth of GaN on graphene. ( c ) Deposition of a stressor layer (Ni). ( d ) Release of GaN from the substrate with a handling tape. ( e ) Transfer of the released GaN/Ni/tape stack on a host substrate. ( f ) Removal of the tape and Ni by thermal release and wet etching, leaving a GaN film on the host substrate. 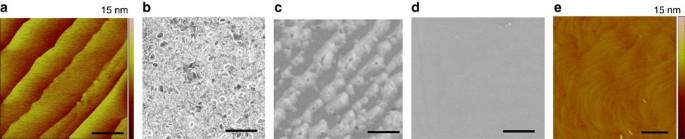Figure 2: Surface morphology of a graphene/SiC substrate and GaN films grown on graphene. (a) AFM image of the surface of a graphitized SiC substrate (scale bar, 10 μm). (b–d) Plan-view SEM images of GaN films grown on graphene (scale bars, 10 μm) by (b) the conventional two-step growth (nucleation at 580 °C and growth at 1,150 °C), (c) one-step growth at 1,100 °C, and (d) modified two-step growth (nucleation at 1,100 °C and growth at 1,250 °C). (e) AFM image of GaN films grown by modified two-step growth showing atomistically smooth surface with RMS roughness of 3 Å (scale bar, 1 μm). Full size image vdWE of planar single crystals on graphene Figure 2a shows the atomic force microscopy (AFM) surface topology of the epitaxial graphene on a SiC substrate after the graphitization. The size of the vicinal steps of the SiC surface was increased by the step bunching during the graphitization [17] . The measured step height and terrace width were 5–10 nm and 5–10 μm, respectively. Continuous films are achievable if GaN nuclei can be preferentially formed first along the periodic step edges and GaN nuclei then advance laterally to coalesce. We performed the growth of GaN on epitaxial graphene by using metalorganic chemical vapour deposition (MOCVD) with following conditions: the conventional two-step growth used for GaN epitaxy on sapphire or SiC (nucleation at 580 °C/growth at 1,150 °C) [15] , [20] , [21] , one-step growth at 1,100 °C and modified two-step growth (nucleation at 1,100 °C/growth at 1,250 °C). Figures 2b–d show plan-view scanning electron microscopy (SEM) images of GaN films grown on graphene by the above three conditions, respectively. The conventional two-step growth (nucleation at 580 °C/growth at 1,150 °C) formed 3D faceted GaN clusters ( Fig. 2b ), whereas one-step growth at 1,100 °C resulted in the formation of continuous GaN stripes (~ 5–10 μm apart) aligned along the SiC vicinal steps ( Fig. 2c ). We speculated that the formation of such faceted clusters from the conventional two-step growth was attributed to the limited atomic mobility at 580 °C together with suppressed nucleation on the graphene surface resulting in the low density of nuclei randomly formed on the terrace [22] , [23] . The formation of stripe patterns from one-step growth at 1,100 °C implies that the increased atomic mobility allows adatoms to nucleate at the energetically favourable step edges [22] , [23] . On the other hand, the modified two-step growth (nucleation at 1,100 °C, growth at 1,250 °C) resulted in the formation of continuous and smooth GaN films ( Fig. 2d ). This could be attributed to the faster lateral growth at an increased growth temperature of 1,250 °C from the GaN nuclei along the periodic terrace edges formed at 1,100 °C (ref. 24 ). A root mean square (RMS) roughness of 3 Å was measured from the surface of GaN formed by the modified two-step growth by using AFM ( Fig. 2e ). Note that no growth occurs when the one-step growth was performed at 1,250 °C due to reduced sticking coefficient (see Supplementary Fig. 1 ). Figure 2: Surface morphology of a graphene/SiC substrate and GaN films grown on graphene. ( a ) AFM image of the surface of a graphitized SiC substrate (scale bar, 10 μm). ( b – d ) Plan-view SEM images of GaN films grown on graphene (scale bars, 10 μm) by ( b ) the conventional two-step growth (nucleation at 580 °C and growth at 1,150 °C), ( c ) one-step growth at 1,100 °C, and ( d ) modified two-step growth (nucleation at 1,100 °C and growth at 1,250 °C). ( e ) AFM image of GaN films grown by modified two-step growth showing atomistically smooth surface with RMS roughness of 3 Å (scale bar, 1 μm). Full size image Detailed structural analysis of the GaN grown on epitaxial graphene was performed using transmission electron microscopy (TEM). As it is known that graphene formed on the SiC surface via Si sublimation retains its unique orientation throughout an entire SiC substrate [16] , [17] , [19] , formation of single-crystalline GaN films was expected if the GaN films were epitaxially grown. The low-magnification TEM image ( Fig. 3a ) shows that a uniform 2.5-μm-thick GaN film was grown on graphene/SiC. The high-resolution TEM (HRTEM) image shows well aligned, ordered crystal lattices of GaN, graphene and 4H-SiC ( Fig. 3b ). 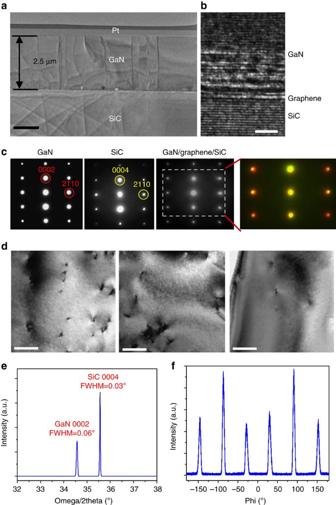Figure 3: TEM and XRD analyses on single crystallinity of GaN films grown on epitaxial graphene. (a) Low-magnification cross-sectional TEM image of 2.5-μm-thick GaN grown on a graphene/SiC substrate (scale bar, 1 μm). (b) HRTEM taken at the interface of GaN/graphene/SiC showing well ordered and aligned crystal lattices of GaN/graphene/SiC (scale bar, 2 nm). (c) Selected area electron diffraction patterns from GaN, SiC, and the interface of GaN/graphene/SiC. All diffraction patterns show the planes of a single-crystalline wurtzite structure. The foil plane vertically aligned with the beam is. The last diffraction pattern is the sum of the GaN and SiC patterns shown. The yellow dots and red dots that appear in a magnified view correspond to SiC and GaN, respectively, indicating excellent alignment of GaN and SiC. (d) Plan-view TEM images of released GaN from the graphene/SiC substrate (scale bar, 0.2 μm). The density of threading dislocations (from left image to right one) is 2.3 × 109cm−2, 1.5 × 109cm−2and 0.4 × 109cm−2. (e) HRXRD omega/2theta scan. Peaks correspond to wurtzite (0002) GaN and (0004) 4H-SiC. (f) HRXRD azimuthal off-axis phi scan. Peaks of GaN (105) at 60° intervals represent the sixfold symmetry of a single-oriented wurtzite crystal. Figure 3c shows selected area electron diffraction patterns taken from GaN and SiC, and across the stack of GaN/graphene/SiC. The diffraction patterns from GaN and SiC indicate planes of a single-crystalline wurtzite structure and they are well aligned (see magnified view in the last image in Fig. 3c to see the alignment). This average proves successful epitaxial growth of GaN on a graphene/SiC substrate. The diffraction from graphene was also observed with a reduced aperture size to 300 nm to focus on the interface, where the graphene patterns appear as streaks due to the lack of plane (see Supplementary Fig. 2 ). To evaluate the crystal quality of the epitaxially grown GaN on graphene, we analysed the defectivity of the GaN film by using plan-view TEM. The average density of threading dislocations over a total inspected area of ~30 μm 2 was approximately 1 × 10 9 cm −2 . Figure 3d shows representative plan-view TEM images. This value is in a good agreement with the density of surface pits in the AFM image ( Fig. 2e ). Notably, this density is in the comparable range with that of AlN-buffer-assisted GaN films grown on the conventional substrates, sapphire or SiC by using MOCVD (5 × 10 8 cm −2 –8 × 10 9 cm −2 ) (refs 25 , 26 , 27 ). Such low dislocation density could be obtained even with ~23% mismatch between GaN and graphene and even without employing AlN buffers, thanks to the successful vdWE of GaN on graphene. Figure 3: TEM and XRD analyses on single crystallinity of GaN films grown on epitaxial graphene. ( a ) Low-magnification cross-sectional TEM image of 2.5-μm-thick GaN grown on a graphene/SiC substrate (scale bar, 1 μm). ( b ) HRTEM taken at the interface of GaN/graphene/SiC showing well ordered and aligned crystal lattices of GaN/graphene/SiC (scale bar, 2 nm). ( c ) Selected area electron diffraction patterns from GaN, SiC, and the interface of GaN/graphene/SiC. All diffraction patterns show the planes of a single-crystalline wurtzite structure. The foil plane vertically aligned with the beam is . The last diffraction pattern is the sum of the GaN and SiC patterns shown. The yellow dots and red dots that appear in a magnified view correspond to SiC and GaN, respectively, indicating excellent alignment of GaN and SiC. ( d ) Plan-view TEM images of released GaN from the graphene/SiC substrate (scale bar, 0.2 μm). The density of threading dislocations (from left image to right one) is 2.3 × 10 9 cm −2 , 1.5 × 10 9 cm −2 and 0.4 × 10 9 cm −2 . ( e ) HRXRD omega/2theta scan. Peaks correspond to wurtzite (0002) GaN and (0004) 4H-SiC. ( f ) HRXRD azimuthal off-axis phi scan. Peaks of GaN (105) at 60° intervals represent the sixfold symmetry of a single-oriented wurtzite crystal. Full size image To determine the macroscopic orientation and the crystal structure, we also performed high-resolution X-ray diffraction (HRXRD) with 2theta/omega scan and azimuthal off-axis phi scans ( Fig. 3e,f , respectively). The XRD spectrum with the 2theta/omega scan represents only two peaks corresponding to single-crystalline wurtzite (0002) GaN and (0004) 4H-SiC ( Fig. 3e ). We have performed multiple scans across the sample and any peaks other than the (0002) GaN peak were not identified. The wider XRD spectrum is shown in Supplementary Fig. 3 . The full-width half maximum of the GaN (0002) peak (=0.06°) is in the similar range to that measured from GaN grown on sapphire or SiC [25] , [26] , [27] (see Supplementary Table 1 ). The phi scan was performed by rotating the sample around its surface normal ( Fig. 3f ). The sixfold symmetry of the diffraction peaks of GaN (105) with 60° intervals indicates that the GaN is a single-crystalline wurtzite phase. Large-area electron backscatter diffraction maps also confirmed the single crystallinity of GaN grown on epitaxial graphene (see Supplementary Fig. 3b ). It should be noted that CVD-grown graphene on Cu foils cannot be employed for obtaining single-crystalline films as the graphene itself is polycrystalline [12] , [13] . Release/transfer of single-crystalline GaN on graphene The TEM and HRXRD analysis conclusively shows that a high-quality single-crystalline GaN film can be grown on an epitaxial graphene surface. Therefore, high technical impact is expected if these high-quality GaN films can be transferred onto the foreign substrates of interest. Release of an overlaying GaN epitaxial film can be initiated either at the GaN/graphene or graphene/SiC interface if the strain energy of the GaN film induced by external stress reaches the van der Waals-bonding energy of the GaN/graphene or graphene/SiC interface. We applied Ni as a stressor layer on GaN because strain energy in GaN can be effectively induced by high-internal stress of Ni (that is, 500 MPa–1 GPa) [18] , [19] . The 2.5-μm-thick GaN film was released from the substrate by a 2-μm-thick Ni stressor as shown in the cross-sectional SEM (XSEM) image ( Fig. 4a ). Thermally released tape was applied on Ni as a handling layer. The interface separation shown in the figure occurred by sample cleaving for the XSEM analysis. Entire GaN epilayer was released from the graphitized substrate with the area of ~1 cm 2 (see Supplementary Fig. 4 )—limited by the size of our MOCVD reactor. In principle, a wafer-scale GaN release is possible. The topology of the released surface of GaN films imaged by AFM ( Fig. 4b ) shows similar terraces to those observed on the surface of an original graphitized SiC substrate ( Fig. 2a ), implying the removal of entire GaN films precisely from the surface of the graphitized SiC substrate. The flat surface of the released GaN layer (RMS roughness of~5 Å measured from AFM image in Supplementary Fig. 5 ) allowed us to bond the released GaN film directly onto (100) Si substrates with a 90-nm SiO 2 layer [28] . As shown in the XSEM image in Fig. 4c , we could achieve the unique structure of GaN on insulator which can be applied for a hybrid GaN and (001) Si co-integration. The formation of excellent bonding of the transferred GaN on SiO 2 was also verified by TEM investigation on the interface (see Supplementary Fig. 6 ). No air gap was detected throughout low magnification and high-resolution TEM analyses. The transferred GaN on insulator shows perfect single-crystalline diffraction patterns indicating no degradation of crystalline quality during the transfer process (see Supplementary Fig. 6 ). 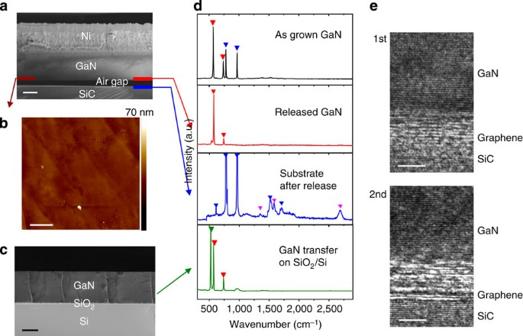Figure 4: Analysis on transferability of GaN from epitaxial graphene and reusability of graphene/SiC substrates. (a) XSEM image of GaN on a graphene/SiC substrate after Ni stressor deposition (scale bar, 1 μm). Separation of the interface between a GaN film and a graphene/SiC substrate is displayed. (b) AFM images taken at the released surface of GaN films (scale bar, 3 μm). The terrace patterns appear as those observed from the graphitized SiC substrate. (c) XSEM image of GaN films directly transferred on a SiO2/Si substrate (scale bar, 1 μm). (d) Raman spectra taken from an as-grown GaN film on a graphene/SiC substrate, released GaN films on the tape, remaining substrate after GaN release and GaN film transferred on SiO2/Si substrate. Red, blue, purple and green inverted triangles correspond to GaN, SiC, graphene and Si, respectively. (e) HRTEM taken at the interface of GaN/graphene/SiC (scale bar, 2 nm). GaN grown on a fresh graphene/SiC substrate is shown on the top, and GaN grown on a reused graphene/SiC substrate after the 1st GaN release is shown on the bottom. They both show comparable crystal order/alignment and graphene still exists on the SiC substrate after GaN release. Figure 4: Analysis on transferability of GaN from epitaxial graphene and reusability of graphene/SiC substrates. ( a ) XSEM image of GaN on a graphene/SiC substrate after Ni stressor deposition (scale bar, 1 μm). Separation of the interface between a GaN film and a graphene/SiC substrate is displayed. ( b ) AFM images taken at the released surface of GaN films (scale bar, 3 μm). The terrace patterns appear as those observed from the graphitized SiC substrate. ( c ) XSEM image of GaN films directly transferred on a SiO 2 /Si substrate (scale bar, 1 μm). ( d ) Raman spectra taken from an as-grown GaN film on a graphene/SiC substrate, released GaN films on the tape, remaining substrate after GaN release and GaN film transferred on SiO 2 /Si substrate. Red, blue, purple and green inverted triangles correspond to GaN, SiC, graphene and Si, respectively. ( e ) HRTEM taken at the interface of GaN/graphene/SiC (scale bar, 2 nm). GaN grown on a fresh graphene/SiC substrate is shown on the top, and GaN grown on a reused graphene/SiC substrate after the 1st GaN release is shown on the bottom. They both show comparable crystal order/alignment and graphene still exists on the SiC substrate after GaN release. Full size image To accurately determine the released interface, we analysed Raman spectra measured from the released surface of GaN films and the surface of the remaining substrate ( Fig. 4d ). The Raman peaks corresponding to graphene was clearly observed from the surface of the post-released SiC substrate, but only GaN peaks were observed from the released film without any peaks corresponding to graphene ( Fig. 4d ). The uniform coverage of graphene on the surface of the post-released SiC substrate was observed by mapping the Raman intensity of graphene 2D peak (see Supplementary Fig. 7 ). The Raman analysis clearly indicates that GaN is released from the surface of graphene instead of being released together with graphene. This result also implies that the bonding energy of GaN/graphene is lower than that of graphene/SiC (~106 meV per atom) [19] . We repeated the sequence of GaN epitaxial growth on the post-released graphene/SiC substrate and the transfer of the GaN layer. Well ordered, aligned GaN crystal lattices on graphene were observed for the first growth and multiple growth of GaN by HRTEM. As an example, we have shown HRTEM images of the GaN/graphene/SiC interface after the first GaN growth and that after the second GaN growth on the graphene/SiC substrate used for the first growth/transfer (see Fig. 4e ). Growth/release of thin-film blue LED on graphene To demonstrate further functionality of our graphene-based single-crystalline multiple-growth/transfer technique, we have performed epitaxial growth of a visible LED stack on a recycled graphene/SiC substrate (previously used ‘three times’). The visible LED stack is composed of three periods of III-nitride multi-quantum wells (InGaN well and GaN barrier) sandwiched between p-GaN and n-GaN layers (see cross-sectional TEM images of a LED stack on graphene/SiC in Fig. 5a,b ). The HRTEM image taken at the GaN/graphene/SiC interface shows well aligned, ordered GaN crystal lattice on a recycled graphene/SiC substrate (see Fig. 5c ). The measured RMS surface roughness was 4 Å. The result of HRXRD also verified the single crystallinity of a InGaN/GaN LED heterostructure on a recycled graphene/SiC substrate as the spectra reveal only two major peaks corresponding to single-crystalline wurtzite (0002) GaN and (0004) 4H-SiC, and satellite peaks corresponding to the multi-quantum wells (see Supplementary Fig. 8 ). The full-width half maximum of the GaN (0002) peak is ~0.06 o , which is same as that of GaN grown on a fresh graphene/SiC substrate. XRD simulation shown in Supplementary Fig. 8 suggests an average indium content of 30% in the 3.5 nm-thick InGaN quantum wells neighbouring the GaN barriers which is required for emission in the blue spectrum. 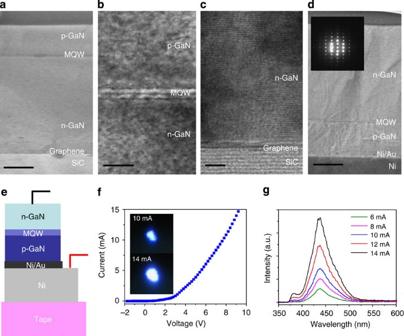Figure 5: Fabrication of GaN blue LED transferred on the tape. (a) Cross-sectional TEM image of LED stacks (p-GaN/MQW/n-GaN) on a graphene/SiC substrate (scale bar, 1 μm). (b) HRTEM image magnified at MQW (scale bar, 100 nm). (c) HRTEM image magnified at a GaN/graphene/SiC interface (scale bar, 5 nm). (d) Cross-sectional TEM image of a released LED stack from a graphene/SiC substrate: n-GaN/MQW/p-GaN/Ni (scale bar, 1 μm). A selected area electron diffraction pattern from p-GaN/MQW/n-GaN is displayed in an inset. (e) Schematic of a transferred visible LED device on the tape. (f)I–Vcharacteristic of a transferred LED stack measured by applying positive bias on Ni and negative bias on n-GaN. The pictures of the LED-emitting blue light are displayed in an inset. (g) Electroluminescence (EL) spectra of a transferred LED stack taken as a function of injection current. Figure 5: Fabrication of GaN blue LED transferred on the tape. ( a ) Cross-sectional TEM image of LED stacks (p-GaN/MQW/n-GaN) on a graphene/SiC substrate (scale bar, 1 μm). ( b ) HRTEM image magnified at MQW (scale bar, 100 nm). ( c ) HRTEM image magnified at a GaN/graphene/SiC interface (scale bar, 5 nm). ( d ) Cross-sectional TEM image of a released LED stack from a graphene/SiC substrate: n-GaN/MQW/p-GaN/Ni (scale bar, 1 μm). A selected area electron diffraction pattern from p-GaN/MQW/n-GaN is displayed in an inset. ( e ) Schematic of a transferred visible LED device on the tape. ( f ) I – V characteristic of a transferred LED stack measured by applying positive bias on Ni and negative bias on n-GaN. The pictures of the LED-emitting blue light are displayed in an inset. ( g ) Electroluminescence (EL) spectra of a transferred LED stack taken as a function of injection current. Full size image To form an electrical contact on the p-GaN, we have deposited thin Ni/Au (5 nm/5 nm) and annealed at 500 °C for 10 min. The entire LED device stack was released by a Ni stressor/handling tape as described earlier (see cross-sectional TEM images of a released LED stack on Ni in Fig. 5d ). A selected area electron diffraction pattern taken from the released LED stack indicates a well-aligned single crystal (see inset of Fig. 5d ). We have directly probed as-released LED stack on Ni/tape as shown in the schematic of the device structure (see Fig. 5e ). A diodic I – V curve was obtained ( Fig. 5f ). The blue light emission from the released LED stack was visually observed (inset of Fig. 5f ) and electroluminescence was recorded ( Fig. 5g ). Electroluminescence spectra confirmed the light emission peaking at λ ≈440 nm which is typical for III-nitride blue LEDs. Our accomplishments, reusing a single graphene/SiC substrate for multiple transfers and direct bonding of GaN on Si substrate enabled by atomistically smooth released interface, are clear contrast to the conventional laser lift-off process, where post-release surface treatment is essential to further repeat the growth/lift-off cycles, and the high roughness of released surface did not allow direct bonding of released layer to the other substrate, it rather requires to apply adhesive to bond the released layers [29] , [30] . In summary, we demonstrated direct vdWE of high-quality single-crystalline GaN on epitaxial graphene/SiC substrates resulting in the average dislocation density of ~1 × 10 9 cm −2 and RMS surface roughness of 3 Å which are within the range to those of AlN-buffer-assisted GaN films grown on the conventional substrates by using MOCVD (5 × 10 8 cm −2 –8 × 10 9 cm −2 ). Entire GaN films on graphene were released and transferred onto arbitrary substrates. The post-released graphene/SiC substrate was reused for multiple growth and transfer cycles of GaN films. Fully functional blue LED was fabricated by performing epitaxial growth of an InGaN/GaN heterostructure on a recycled graphene/SiC substrate followed by release of the heterostructure. Formation of epitaxial graphene An epitaxial graphene with a single-crystalline orientation is grown on the Si face of a (0001) 4H-SiC wafer via multistep annealing, first in H 2 gas for surface etching and vicinalization, and then in Ar for graphitization at 1,575 °C. Epitaxial growth of GaN on graphene/SiC Epitaxial growth of GaN films on the graphene/SiC substrate was performed in a horizontal flow, low-pressure MOCVD reactor. A graphene/SiC substrate was baked under H 2 for >15 min at >1,100 °C for cleaning the surface. The deposition of a 2.5-μm-thick GaN layer was immediately followed at 200 mbar. Trimethylgallium, ammonia and hydrogen were used as a Ga source, nitrogen source and carrier gas, respectively. A modified two-step growth was employed to obtain flat GaN epitaxial films on the epitaxial graphene. The first step was carried out at a growth temperature of 1,100 °C for few minutes where guided nucleation at terrace edges was promoted. The second growth step was carried out at an elevated temperature of 1,250 °C to promote the lateral growth. Vertical GaN growth rate was around 20 nm min −1 . Release/transfer of epitaxial GaN on graphene The Ni stressor was deposited in the evaporator at a vacuum level of 1 × 10 −5 Torr. GaN was then completely released using the thermally released tape-handling layer. The remaining graphene/SiC substrate is dipped into FeCl 3 -based solution to completely remove Ni residue for the next GaN regrowth. The released GaN film is transferred onto the Si wafer coated with 90-nm SiO 2 by pressing down the stack of layers, followed by the removal of the thermal tape by annealing above the release temperature of 90 °C, and then etching the Ni film in a FeCl 3 -based solution. The above steps were repeated for multiple transfers. TEM sample preparation For the preparation of a plan-view TEM sample, a released stack (thermal release tape/Ni/GaN) was fixed to a copper grid. Then, the tape was thermally released followed by removal of Ni via Argon ion milling. The area imaged for the defectivity is the top 200 nm of GaN material. Growth of LED on graphene The material growth for the LED was carried out in a MOCVD. The first n-GaN was grown by using modified two-step growth at 1,100—1,250 °C followed by growing three periods of InGaN/GaN active layer at ~700 °C. The active layer was then capped with a p-GaN layer deposited at 1,050 °C. The LED structure was later annealed at 1,000 °C for 30 s under N 2 ambient for carriers in the p-type material. How to cite this article: Kim, J. et al . Principle of direct van der Waals epitaxy of single-crystalline films on epitaxial graphene. Nat. Commun. 5:4836 doi: 10.1038/ncomms5836 (2014).